Natural variation inBnaA9.NF-YA7contributes to drought tolerance inBrassica napusL Rapeseed (Brassica napus) is one of the important oil crops worldwide. Its production is often threatened by drought stress. Here, we identify a transcription factor (BnaA9.NF-YA7) that negatively regulates drought tolerance through genome-wide association study in B. napus . The presence of two SNPs within a CCAAT cis element leads to downregulation of BnaA9.NF-YA7 expression. In addition, the M63I (G-to-C) substitution in the transactivation domain can activate low level expression of BnaA4.DOR , which is an inhibitory factor of ABA-induced stomatal closure. Furthermore, we determine that Bna.ABF3/4 s directly regulate the expression of BnaA9.NF-YA7 , and BnaA9.NF-YA7 indirectly suppresses the expression of Bna.ABF3/4 s by regulation of Bna.ASHH4s . Our findings uncover that BnaA9.NF-YA7 serves as a supplementary role for ABA signal balance under drought stress conditions, and provide a potential molecular target to breed drought-tolerant B. napus cultivars. Brassica napus L. ( B. napus ; AACC, 2 n = 38), an amphidiploid species formed by the natural hybridization of Brassica rapa (AA, 2 n = 20) and Brassica oleracea (CC, 2 n = 18) [1] , is an excellent source of edible vegetable oil and protein and constitutes the second-largest vegetable oil source in the world [2] , [3] , [4] . However, drought stress has a major limiting impact on its production and yield stability [5] , and drought accounts for at least a 30% yield loss in B. napus every year [6] . Therefore, exploring the mechanisms by which B. napus responds to drought stresses and how the resistance of B. napus to drought stress may be improved has great significance. To date, some drought-responsive genes, including LEA3 and VOC (which alter drought tolerance and lipid accumulation [2] ), BnaYUC6a (which is associated with high auxin production and drought tolerance [7] ), BnaA6.RGA (which enhances drought tolerance [8] ), and BnaA01.CIPK6 (which confers drought tolerance [9] ), have been cloned and functionally characterized in B. napus . However, the molecular regulation of drought tolerance in B. napus is largely unknown. Nuclear factor-Y (NF-Y), also known as heme activator protein (HAP) or CCAAT-binding factor (CBF), is a sequence-specific transcription factor with nonspecific DNA-binding nucleosome properties that is ubiquitous in eukaryotes, and is composed of NF-YA, NF-YB, and NF-YC subunits [10] , [11] . The three subunits can form a heterotrimeric complex and bind to the downstream gene CCAAT-box, one of the sequence elements most frequently found in eukaryotic promoters, and regulate its expression [11] . In recent years, many studies have found that NF-Y transcription factors in plants play an important role in plants’ ability to cope under various abiotic stresses, including drought stress [12] , [13] , [14] , [15] . From a functional viewpoint, NF-Y is considered a facilitator of TF binding and an architectural promoter organizer [11] . Furthermore, NF-Y complex binding to DNA is also important for the establishment of histone posttranslational modifications (PTMs) through the recruitment of relevant enzymes [16] . Here, we report that an NF-YA subunit, BnaA9.NF-YA7, is involved in B. napus drought tolerance at the seedling stage. Two SNPs in the promoter and a nonsynonymous substitution (M63I) in BnaA9.NF-YA7 confer B. napus drought tolerance by regulating the ABA signal transduction pathway via feedback inhibition of the expression of BnaABF3/4s -related genes. Natural variation in BnaA9.NF-YA7 is associated with drought tolerance Further mining of previously published data [17] showed that BnaA9.NF-YA7 is associated with the germination percentage (GP) and germination index (GI) under drought stress and that BnaA9.NF-YA7 is upregulated by drought stress under repeated drought-rewatering cycles (Supplementary Fig. 1 ). To investigate functional allelic variations in the BnaA9.NF-YA7 locus, 48 variation sites covering the BnaA9.NF-YA7 promoter (2 kb) and gene were identified based on previously published resequencing data [18] (Supplementary Data 1 ). Candidate gene association analysis was performed for GP and GI using 181 inbred lines from the resequencing population and five SNPs were identified above the suggestive significance threshold of association ( P < 0.01; Supplementary Fig. 2a, b ). Moreover, GWAS performed in this natural-variation population for water holding capacity (WHC) under drought stress using a mixed linear model approach identified ten associated loci meeting the threshold for suggestive evidence of association ( P < 1.7 × 10 −7 ), of which the most significant signal (S9_19159584) was located within the third exon of BnaA9.NF-YA7 (Fig. 1a and Supplementary Fig. 2c ). Fig. 1: Natural variation in BnaA9.NF-YA7 is associated with drought tolerance. a Regional Manhattan plot of the BnaA9.NF-YA7 genomic region on chromosome A09. The 2-Mb genomic region on either side of the most significant SNP is shown. The lead SNP is shown with a red dot, and the other SNPs are colored according to their LD ( r 2 value) with the lead SNP. b Pairwise LD estimates for BnaA9.NF-YA7 gene locus. The green arrows denote the significantly associated SNP in BnaA9.NF-YA7 . c The different varieties from five haplotypes survived after 14 days of drought treatment followed by 5 days of rewatering. Scale bars = 5 cm. d Comparison of survival rates among accessions of the five haplotypes. Values are means ± SD (Hap1: n = 27 accessions examined over ten independent experiments; Hap2: n = 188 accessions examined over ten independent experiments; Hap3: n = 14 accessions examined over ten independent experiments; Hap4: n = 9 accessions examined over ten independent experiments; Hap5: n = 11 accessions examined over ten independent experiments;). The lowercase letters indicate significant differences ( P < 0.05, one-way ANOVA followed by two-tailed Fisher’s least significant difference (LSD) test). e Bean plot showing the water holding capacity of accessions from two alleles. P values were calculated with the two-tailed Student’s t -test (C: n = 21 accessions; G: n = 184 accessions). f The level of population differentiation ( F ST ) across chromosome A09 between B. napus and B. rapa . g Expression levels of BnaA9.NF-YA7 in five haplotypes under 0.2 M d -mannitol treatment. The values are means ± SD ( n = 3 biological replicates). Asterisks indicate statistically significant differences between Hap3 and Hap4 interaction based on two-tailed Student’s t -test (*** P < 0.001 and P = 4.18 × 10 −5 , 3.50 × 10 −4 , 8.85 × 10 −5 , and 4.20 × 10 −4 at the time points of 3, 6, 12, and 24 h). h Expression levels of BnaA9.NF-YA7 in Hap3 and Hap4 under 15% PEG treatment. The values are means ± SD ( n = 3 biological replicates). Asterisks indicate statistically significant differences between Hap3 and Hap4 interaction based on two-tailed Student’s t -test (** P < 0.01, *** P < 0.001, and P = 1.78 × 10 -5 , 5.92 × 10 −4 , 8.71 × 10 −5 , 3.70 × 10 −3 , and 5.78 × 10 −6 at the time points of 3, 6, 24, 48, and 72 h). n.s. not significant. Source data are provided as a Source Data file. Full size image Interestingly, S9_19159584 (G-to-C), in which the methionine at the 63rd position was changed to isoleucine (M63I) in BnaA9.NF-YA7 , was in strong linkage disequilibrium (LD) with the SNPs within the promoter region (Fig. 1b ). The 608 rapeseed genotypes were classified into five haplotype groups (Supplementary Fig. 2d ), based on the SNPs within BnaA9.NF-YA7 (MAF ≥0.03), and physiologic index analysis showed significant differences among different haplotypes, especially Hap3 and Hap4 (Fig. 1c, d and Supplementary Fig. 2e–h ). Moreover, the accessions with the C allele (Hap1 and Hap4, referred to as BnaA9.NF-YA7 C ) had a higher WHC than the accessions with the G allele (referred to as BnaA9.NF-YA7 G ) after drought treatment (Fig. 1e and Supplementary Fig. 2i ). However, no mutation sites significantly associated with drought tolerance were found in another homolog BnaC5.NF-YA7 in B. napus (Supplementary Fig. 2c ). Together, these results suggest the genetic variation in BnaA9.NF-YA7 could be involved in the drought tolerance of B. napus . Next, we performed multiple sequence alignments and phylogenetic tree analysis of the BnaA9.NF-YA7 protein sequence. Surprisingly, the genotypes of Bra.NF-YA7 , Bol.NF-YA7 and BnaC5.NF-YA7 at position 63 were consistent with BnaA9.NF-YA7 C (Supplementary Fig. 3a ), and BnaA9.NF-YA7 C was evolutionarily closer to Bra.NF-YA7 (Supplementary Fig. 3b ), indicating that only 10% (52/608) of the C alleles in B. napus were from ancestral species. Nevertheless, the M63I substitution did not change the tertiary structure of the protein (Supplementary Fig. 3c ). Several BnaA9.NF-YA7 fragments were designed based on the domain structure of BnaA9.NF-YA7 (Supplementary Fig. 3d ). The Y2H (self-activation) assay and dual-luciferase reporter assay showed that BnaA9.NF-YA7 had different transcriptional activation abilities in Hap3 and Hap4 (Supplementary Fig. 3e–h ), and the M63I substitution occurred in a Pro-rich transcriptional activation domain (Supplementary Fig. 3a ). Unlike the Hap1 varieties, the Hap4 members were clustered in a small subgroup of the semi-winter ecotype (Supplementary Fig. 4a ). The highest F ST levels appeared at the site in BnaA9.NF-YA7 and its flank but not in BnaC5.NF-YA7 (Fig. 1f and Supplementary Fig. 4b ), suggesting that BnaA9.NF-YA7 possibly underwent strong selection during the domestication stage. BnaA9.NF-YA7 was greatly induced by drought and abscisic acid Under nonstress conditions, higher levels of BnaA9.NF-YA7 transcripts were found in embryos, leaves, and seeds compared with other tissues, similar to the result for BnaC5.NF-YA7 (Supplementary Fig. 5a ). BnaA9.NF-YA7 expression was significantly induced by drought stress, and the expression level of Hap3 was significantly higher than that of Hap4 (Supplementary Fig. 5b ). The same phenomenon occurred under osmotic stress simulated by 0.2 M d -mannitol and 15% PEG, with a negative correlation between survival rate and expression level, which was almost the same as the result under drought treatment (Fig. 1g, h and Supplementary Fig. 5c, d ). Unexpectedly, the expression level of Hap1 was also higher than that of Hap4 (Fig. 1g ). Moreover, the expression of BnaC5.NF-YA7 was also induced by drought, but the level of BnaC5.NF-YA7 was not significantly different among the five haplotypes (Supplementary Fig. 5e ). Compared to the unaltered transcripts in water-treated leaves (Supplementary Fig. 6a ), the expression of BnaA9.NF-YA7 was upregulated by H 2 O 2 , ABA, and SNP (sodium nitroprusside, nitric oxide producer) treatment, and there were also differences between Hap3 and Hap4 (Supplementary Fig. 6b–d ). Likewise, the expression of BnaA9.NF-YA7 was significantly induced after dehydration treatment (Supplementary Fig. 6e ). Upregulation of BnaA9.NF-YA7 expression by ABA treatment and induction of BnaA9.NF-YA7 expression was suppressed by pretreatment with FLU (fluridone, an inhibitor of ABA biosynthesis) in detached leaves, suggesting that ABA was an essential signal for dehydration-induced transcription of BnaA9.NF-YA7 (Supplementary Fig. 6f ). These findings indicated that BnaA9.NF-YA7 is responsive to drought stress and ABA signaling. BnaA9.NF-YA7 negatively regulates B. napus drought tolerance To confirm the function of BnaA9.NF-YA7 , we generated transgenic B. napus plants (Supplementary Fig. 7 ). The results of drought tolerance evaluation showed that most of the knockout and RNAi seedlings survived after a 5-day recovery because of increased leaf water holding capacity and decreased water loss rate and transpiration rate (Fig. 2a–e and Supplementary Fig. 8a–e ). A similar result was also observed for germination under d -mannitol treatment; the knockout seedlings exhibited increased root length and hypocotyl length, but the BnaA9.NF-YA7-OE lines had shorter roots and hypocotyls than the WT (Supplementary Fig. 8f–h ). These results demonstrate that BnaA9.NF-YA7 functions as a negative regulator of B. napus drought tolerance. Furthermore, we noted that there was no significant difference in drought tolerance between the BnaA9.NF-YA7 C and BnaA9.NF-YA7 G -overexpressing transgenic lines (Fig. 2f ), but the drought tolerance of Hap3 could be slightly enhanced by the site-directed mutation M63I (Supplementary Fig. 8i, j ). Fig. 2: BnaA9.NF-YA7 negatively regulates B. napus drought tolerance by increasing stomatal conductance and the transpiration rate. a Phenotype of B. napus seedlings grown in plastic pots under well-watered, drought stress, or rewatering conditions. Bar = 5 cm. b , c The survival rate ( b ) and water holding capacity ( c ) of overexpression and knockout lines were compared with those of WT. The values are means ± SD ( n = 50 plants examined over ten independent experiments in ( b ) and n = 10 biologically independent experiments in ( c ). P values were calculated with the two-tailed Student’s t -test. d , e Infrared thermal images show the wild-type and BnaA9.NF-YA7 transgenic lines ( d ) and the corresponding leaf surface temperature ( e ) before drought treatment. The values are means ± SD ( n = 10 biologically independent experiments). P values were calculated with the two-tailed Student’s t -test. Bar = 5 cm. f The drought tolerance was not significantly different between the 35S:BnaA9.NF-YA7 C and 35S:BnaA9.NF-YA7 G transgenic lines. Bar = 1 cm. g Phenotype of stomata between wild-type and BnaA9.NF-YA7 transgenic lines under well-watered conditions. Bar = 10 μm. h – k Comparison of stomatal length ( h ), stomatal width ( i ), stomatal density ( j ), and stomatal index ( k ) between wild-type and BnaA9.NF-YA7 transgenic lines. The values are means ± SD ( n = 50 biological replicates in ( h , i ); n = 10 biological replicates in ( j , k ). l , m Stomatal conductance ( l ) and transpiration rate ( m ) before and after ABA treatment. Values are mean ± SD ( n = 5 biologically independent experiments). The lowercase letters indicate significant differences ( P < 0.05, One-way ANOVA followed by two-tailed LSD test). n Phenotype of different genotypes grown on half-strength MS phytoagar medium containing 0, 1, or 5 μM ABA for 14 days under LD conditions. White bars = 2 cm. o , p Quantification of root length ( o ) and hyp o cotyl length ( p ) after 14 days of ABA treatment. The values are means ± SDs ( n = 10 biological replicates). P values were calculated with the two-tailed Student’s t -test. q Infrared thermal images of WT and BnaA9.NF-YA7-OE plants before and after ABA treatment. White bars = 1 cm. Source data are provided as a Source Data file. Full size image In comparison with wild-type plants, the aaCC ( BnaA9.NF-YA7 knockout) and aacc ( BnaA9.NF-YA7/BnaC5.NF-YA7 double knockout) lines had smaller stomata and lower stomatal density (Fig. 2g–k ), exhibiting lower stomatal conductance and transpiration rate under nonstress conditions (Fig. 2l, m ). Conversely, overexpressing BnaA9.NF-YA7 led to increased stomatal conductance and transpiration rate compared with those of the WT, but significant differences were not found among these transgenic plants after ABA treatment (Fig. 2l, m ). Additional confirmation was obtained by using infrared thermal imaging to visualize the surface temperature of detached leaves, in which the leaf surface temperature of the overexpression lines was lower due to more water loss than that of the WT and knockout lines before dehydration treatment (Supplementary Fig. 8a and Supplementary Fig. 9a, b ), while that of the knockout line was slightly higher than that of the WT after 2 h of dehydration (Supplementary Fig. 9c ). ABA treatment significantly inhibited root and hypocotyl growth in all genotypes (Fig. 2n ), and the inhibition degree significantly increased in BnaA9.NF-YA7-OE plants compared to the WT and BnaA9.NF-YA7-KO lines (Fig. 2o, p ), indicating that overexpression of BnaA9.NF-YA7 increased ABA sensitivity. However, the percentage of closed stomata was significantly lower in BnaA9.NF-YA7-OE (19.68%) compared to WT (52.50%) or BnaA9.NF-YA7-KO (62.87%) leaves after drought treatment (Supplementary Fig. 9d, e ), similar to the result for ABA treatment (Fig. 2q ). These results indicated that BnaA9.NF-YA7 negatively regulates drought tolerance by increasing stomatal conductance and the transpiration rate. CCAAT-box variation affects the expression level of BnaA9.NF-YA7 GUS activity was clearly detected in all tissues and organs except for the root tip with different degrees of expression; in particular, GUS staining was more vasculature-specific in seedlings (Supplementary Fig. 10 ). In 2-week-old plants, GUS activity and GUS expression levels in leaves were significantly different between Hap3 and Hap4 under abiotic stress (Fig. 3a–c ). To accurately identify the specific mutation sites that led to the differences in Hap3 and Hap4 expression levels, we conducted promoter truncation analysis and found that the ABRE, CCAAT-box, and motif_sequence were the core cis-acting elements of the BnaA9.NF-YA7 promoter (Fig. 3d ), but the presence of two SNPs led to the CCAAT-box deletion in only Hap4, not in the other haplotypes (Fig. 3e and Supplementary Fig. 11 ). These findings provide strong evidence that CCAAT-box variation is directly involved in the difference in BnaA9.NF-YA7 transcript levels between Hap4 and other haplotypes (including Hap1). Fig. 3: CCAAT-box variation affects the expression level of BnaA9.NF-YA7 . a GUS staining of ProBnaA9.NF-YA7 Hap3 :GUS and ProBnaA9.NF-YA7 Hap4 :GUS seedlings under normal conditions and 5 mM PEG, 0.5 µM ABA, and 0.2 M d -mannitol treatment. Scale bars, 2 mm, 5 mm or 500 µm. b , c GUS enzyme activity ( b ) and GUS expression level ( c ) between ProBnaA9.NF-YA7 Hap3 :GUS and ProBnaA9.NF-YA7 Hap4 :GUS seedlings under normal conditions. The values are means ± SD ( n = 3 biological replicates). P values were calculated with the two-tailed Student’s t -test. d GUS enzyme activity of transgenic plants after fusion of the GUS reporter gene with BnaA9.NF-YA7 promoter fragments of different lengths. The values are means ± SDs ( n = 3 biologically independent experiments). D1–D11 indicates BnaA9.NF-YA7 promoter fragments of different lengths. The lowercase letters indicate significant differences ( P < 0.05, one-way ANOVA followed by a two-tailed LSD test). e SNP variation of the CCAAT-box within the promoter region of BnaA9.NF-YA7 between Hap4 and the other Haps. The sequences on the red lines are the target site. The red characters indicate substitutions. f Schematic diagram showing the constructs used in the transient transactivation analysis. g NF-Y trimers can activate the expression of BnaA9.NF-YA7 , and the CCAAT-box variation affects the expression level of BnaA9.NF-YA7 between Hap3 and Hap4. The values are means ± SD ( n = 3 biologically independent experiments). P values were calculated with the two-tailed Student’s t- test. Source data are provided as a Source Data file. Full size image To confirm this hypothesis, expression analysis and clustering of all NF-Y subunits (41 putative BnaNF-YA, 43 putative BnaNF-YB, and 18 putative BnaNF-YC subunits) were performed under repeated drought-rewatering treatment, and the NF-YA/YB/YC subunits within the B2 subgroup to which BnaA9.NF-YA7 belongs were selected for interaction analysis (Supplementary Fig. 12a ). Y2H and BiFC assays detected interactions between BnaA9.NF-YB2 and BnaA6.NF-YC9, BnaA9.NF-YB2, and BnaC5.NF-YC9 (Supplementary Fig. 12b, c ), and the BnaA9.NF-YB2/BnaA6.NF-YC9 dimer formed a trimer with BnaA6.NF-YA5 and BnaC5.NF-YA9 by yeast three-hybrid (Y3H) analysis (Supplementary Fig. 12d ). Next, transient dual-luciferase assays were performed in Arabidopsis protoplasts. When co-transforming with an empty effector construct, the LUC activity of the Hap3 reporter was not different from that of the Hap4 reporter (Fig. 3f, g ). Co-expression of BnaA9.NF-YB2/BnaA6.NF-YC9 with BnaA6.NF-YA5 induced LUC activity in both the Hap3 and Hap4 reporters, similar to BnaA9.NF-YB2/BnaC5.NF-YC9 with BnaC5.NF-YA9, whereas the Hap4 reporter exhibited lower LUC activity than the Hap3 reporter ( P < 0.001, Fig. 3f, g ), which explained the difference in expression levels between Hap3 and Hap4. In addition, we found that BnaA9.NF-YA7 can induce higher LUC activity in the Hap3 reporter than in Hap4, and BnaA9.NF-YA7 G induced higher LUC activity than BnaA9.NF-YA7 C , which further confirms that the M63I substitution is in the transcriptional activation region. BnaABF3/4s directly regulate the activity of BnaA9.NF-YA7 To explore the upstream regulators that regulate BnaA9.NF-YA7 expression under drought stress, we screened for proteins that interact with D5 (a fragment of the promoter of BnaA9.NF-YA7 , Fig. 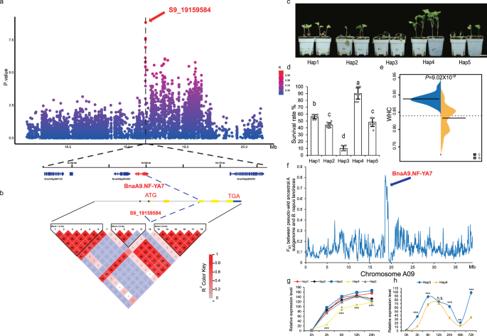Fig. 1: Natural variation inBnaA9.NF-YA7is associated with drought tolerance. aRegional Manhattan plot of theBnaA9.NF-YA7genomic region on chromosome A09. The 2-Mb genomic region on either side of the most significant SNP is shown. The lead SNP is shown with a red dot, and the other SNPs are colored according to their LD (r2value) with the lead SNP.bPairwise LD estimates forBnaA9.NF-YA7gene locus. The green arrows denote the significantly associated SNP inBnaA9.NF-YA7.cThe different varieties from five haplotypes survived after 14 days of drought treatment followed by 5 days of rewatering. Scale bars = 5 cm.dComparison of survival rates among accessions of the five haplotypes. Values are means ± SD (Hap1:n= 27 accessions examined over ten independent experiments; Hap2:n= 188 accessions examined over ten independent experiments; Hap3:n= 14 accessions examined over ten independent experiments; Hap4:n= 9 accessions examined over ten independent experiments; Hap5:n= 11 accessions examined over ten independent experiments;). The lowercase letters indicate significant differences (P< 0.05, one-way ANOVA followed by two-tailed Fisher’s least significant difference (LSD) test).eBean plot showing the water holding capacity of accessions from two alleles.Pvalues were calculated with the two-tailed Student’st-test (C:n= 21 accessions; G:n= 184 accessions).fThe level of population differentiation (FST) across chromosome A09 betweenB. napusandB. rapa.gExpression levels ofBnaA9.NF-YA7in five haplotypes under 0.2 Md-mannitol treatment. The values are means ± SD (n= 3 biological replicates). Asterisks indicate statistically significant differences between Hap3 and Hap4 interaction based on two-tailed Student’st-test (***P< 0.001 andP= 4.18 × 10−5, 3.50 × 10−4, 8.85 × 10−5, and 4.20 × 10−4at the time points of 3, 6, 12, and 24 h).hExpression levels ofBnaA9.NF-YA7in Hap3 and Hap4 under 15% PEG treatment. The values are means ± SD (n= 3 biological replicates). Asterisks indicate statistically significant differences between Hap3 and Hap4 interaction based on two-tailed Student’st-test (**P< 0.01, ***P< 0.001, andP= 1.78 × 10-5, 5.92 × 10−4, 8.71 × 10−5, 3.70 × 10−3, and 5.78 × 10−6at the time points of 3, 6, 24, 48, and 72 h). n.s. not significant. Source data are provided as a Source Data file. 3d ) using a Y1H assay with a cDNA library prepared from drought-treated B. napus leaves (Supplementary Table 1 ). Among the potential regulatory genes, BnaABF3/4s were particularly interesting because of the upregulated expression of BnaA9.NF-YA7 induced by ABA. Both the Y1H assay and electrophoretic mobility shift assay (EMSA) showed that BnaC7.ABF3 and BnaA3.ABF4 bound the ABRE sites in the BnaA9.NF-YA7 promoter in vitro (Fig. 4a–d ). Furthermore, ChIP‒qPCR identified enrichment in the fragment spanning the ABRE sites in the BnaA9.NF-YA7 promoter (Fig. 4e–g ). We thus believed it was possible that BnaC7.ABF3 and BnaA3.ABF4 regulated the expression of BnaA9.NF-YA7 under ABA induction. Fig. 4: BnaABF3/4 s directly upregulates the transcription of BnaA9.NF-YA7 . a Y1H indicated that BnaABF3/4 s could bind the BnaA9.NF-YA7 promoter. b – d EMSA showed that BnaC7.ABF3 ( c ) and BnaA3.ABF4 ( d ) could bind the ABRE sites in the BnaA9.NF-YA7 promoter. The biotin-labeled probes are indicated in ( b ). e The fragments used in ChIP‒qPCR. f , g ChIP‒qPCR identified BnaC7.ABF3 ( f ) and BnaA3.ABF4 ( g ) as significantly enriched in the fragment containing the ABRE sites in the BnaA9.NF-YA7 promoter. Fold enrichments in ( f ) and ( g ) were calculated relative to input. The values are means ± SD ( n = 3 biological replicates). h Schematic diagram showing the constructs used in the transient transactivation analysis. i BnaC7.ABF3 and BnaA3.ABF4 activates BnaA9.NF-YA7 independently or in the form of dimers. The values are means ± SDs ( n = 6 biologically independent experiments). The lowercase letters indicate significant differences ( P < 0.05, One-way ANOVA followed by two-tailed LSD test). Source data are provided as a Source Data file. Full size image A previous study suggested that AtABF3 and AtABF4 interact in Arabidopsis [19] . We tested for an interaction between the BnaC7.ABF3 and BnaA3.ABF4 proteins before further determining how this circuit was regulated, and both the Y2H assay and BiFC assay showed that there was a physical interaction between BnaC7.ABF3 and BnaA3.ABF4 (Supplementary Fig. 13a, b ). Transient expression assays showed that overexpressing BnaC7.ABF3 or BnaA3.ABF4 alone induced the LUC activity of both the Hap3 and Hap4 reporters, and co-expression of BnaC7.ABF3 with BnaA3.ABF4 further induced the activity of the two reporters, whereas there was no significant difference in LUC activity between the Hap3 and Hap4 reporters (Fig. 4h, i ). To further determine the regulatory relationship of BnaA9.NF-YA7 with BnaC7.ABF3 , we examined their expression in the leaves of BnaC7.ABF3 transgenic plants. The expression level of BnaA9.NF-YA7 was significantly increased in the BnaC7.ABF3-OE lines, but the transcript was repressed in the BnaC7.ABF3-RNAi lines even after ABA treatment, whereas the expression of BnaC7.ABF3 was unaltered in the BnaA9.NF-YA7-RNAi line (Supplementary Fig. 13c ). Together, these data clearly indicate that BnaA9.NF-YA7 functions downstream of BnaABF3/4s . Identification of stress-related genes controlled by BnaA9.NF-YA7 To understand the different molecular mechanisms regulated by BnaA9.NF-YA7 under drought stress, we compared the transcriptomes of leaves from drought-stressed 4-week-old Hap3 and Hap4 plants using RNA-Seq. The DEGs were stratified into hormone-mediated signaling pathway, regulation of jasmonic acid-mediated signaling pathway, and response to abiotic stimulus (Supplementary Fig. 14a and Supplementary Data 2 ), indicating that the difference between Hap3 and Hap4 is involved in a diverse range of biological processes and molecular functions. Moreover, we conducted RNA-Seq analysis using WT, BnaA9.NF-YA7-OE, and BnaA9.NF-YA7-KO (aaCC, aacc, and AAcc homozygous mutant plants) seedlings after drought stress to explore the genome-wide transcriptional landscape dictated by BnaA9.NF-YA7 . Through gene ontology (GO) analysis, these DEGs were found to be enriched in “response to water deprivation”, “response to abscisic acid”, “response to abiotic stimulus”, and “response to osmotic stress” (Supplementary Fig. 14b, c and Supplementary Data 3, 4 ). Notably, Venn diagram analysis showed that aaCC and AAcc shared 4706 DEGs (Supplementary Fig. 14d ), indicating that, to a great extent, BnaA9.NF-YA7 and BnaC5.NF-YA7 share similar downstream targets and plays largely redundant roles during these different biological processes. However, we also found that the DEGs specifically regulated by BnaA9.NF-YA7 or BnaC5.NF-YA7 were stratified into different sets of biological processes (Supplementary Fig. 14e ), suggesting that BnaA9.NF-YA7 and BnaC5.NF-YA7 may have distinct roles due to functional differentiation. To better identify direct BnaA9.NF-YA7-binding motifs and target genes in B. napus , a ChIP-Seq assay was performed. A total of 4210 and 24,578 binding peaks were identified and associated with 3939 and 15,579 neighboring genes in the CK (normal conditions as control) and DS (drought stress) sets, respectively (Supplementary Fig. 15a and Supplementary Data 5 ). As expected, the canonical NF-Y-binding motif CCAAT was identified in the center of the ChIP-Seq peaks, but there were significant differences in the flanking sequence of the CCAAT motif identified between CK and DS (Supplementary Fig. 15b ). The target genes of BnaA9.NF-YA7 identified by ChIP-Seq were compared with the DEGs identified by RNA-Seq (Fig. 5a ). In this way, common DEGs that were upregulated in BnaA9.NF-YA7-OE and downregulated in BnaA9.NF-YA7-KO or downregulated in BnaA9.NF-YA7-OE and upregulated in BnaA9.NF-YA7-KO were then extracted as high-confidence genes regulated by BnaA9.NF-YA7 . A total of 1004 and 951 genes from the intersection of the Venn diagram were enriched in alpha-linolenic acid metabolism, biosynthesis of secondary metabolites, plant hormone signal transduction, and MAPK signaling pathway-plant (Supplementary Fig. 15c ). Fig. 5: BnaA9.NF-YA7 directly targets BnaABF3s . a Venn diagrams of the DEGs from transcriptomes and target genes of ChIP-Seq. b Genome browser view of normalized ChIP-Seq tags from the ChIP-Seq data and normalized RNA-Seq tags from the RNA-Seq data for BnaA9.NF-YA7 , showing examples of BnaC7.ABF3 bound by BnaA9.NF-YA7 TFs. c , d GST pull-down ( c ) and co-immunicprecipitation assays ( d ) testing the interactions among BnaA9.NF-YA7 and BnaA9.NF-YB2/BnaA6.NF-YC4 in vitro and in vivo. e EMSA showing that NF-Y containing BnaA9.NF-YA7 could bind the CCAAT sites in the BnaABF3s promoter. Labeled probes containing the CCAAT element (Supplementary Fig. 18d , near TSS or within the coding region) were synthesized and labeled with biotin. The cold (unlabeled) probe and mutated CCAAT element (labeled) were used as a competitor and mutant probes, respectively. f Phenotype of B. napus seedlings grown in plastic bins (length × width × depth = 32 × 20 × 10 cm) under well-watered, drought stress, or rewatering conditions. WT indicates wild-type ZS 11 plants, DO indicates BnaA9.NF-YA7 and BnaC7.ABF3 double overexpression lines Bar = 2 cm. g The survival rate of BnaA9.NF-YA7-OE, BnaC7.ABF3-OE, and double overexpression lines were compared with that of the WT. The values are means ± SD ( n = 50 plants examined over ten independent experiments). h Transpiration rate of BnaA9.NF-YA7-OE, BnaC7.ABF3-OE, and double overexpression lines were compared with WT under normal conditions. The values are means ± SD ( n = 3 biological replicates). The lowercase letters indicate significant differences ( P < 0.05, one-way ANOVA followed by a two-tailed LSD test). Source data are provided as a Source Data file. Full size image BnaA9.NF-YA7 directly targets BnaABF3/4s Notably, the genes involved in plant hormone signal transduction included ABA-responsive element (ABRE)-binding factors (ABFs) (i.e., BnaABF2s , BnaABF3s , and BnaABF4s ), which function redundantly as master regulators of ABA signaling in response to drought and osmotic stresses [20] , and these genes were downregulated in the BnaA9.NF-YA7-OE lines, especially BnaABF3s and BnaC1.ABF4 (Supplementary Data 6 ). BnaAn.ABF3 , BnaC1.ABF3 , BnaC7.ABF3 , and BnaC1.ABF4 were determined to have two to three potential binding sites containing CCAAT-box motifs in the promoter and coding regions (Fig. 5b and Supplementary Fig. 16a ). In general, the ChIP‒qPCR values were consistent with the ChIP-Seq results (Supplementary Fig. 16b ). Y2H and BiFC assays were performed to identify the BnaNF-YB/YC dimer that can interact with BnaA9.NF-YA7 to form a trimer (Supplementary Fig. 17a, b ), and each of these dimers were individually fused to GAL4 DNA-BD in a Y3H system to assess their potential interaction with the BnaA9.NF-YA7 protein (Supplementary Fig. 17c, d ). Y3H, α-galactosidase activity, and FRET (fluorescence resonance energy transfer) assays showed that BnaA9.NF-YB2 and BnaA6.NF-YC4 could differentially form a trimer complex with BnaA9.NF-YA7 in Hap3 (representative BnaA9.NF-YA7 G ) compared to that in Hap4 (representative BnaA9.NF-YA7 C ) (Supplementary Fig. 18a–c ). Both the GST pull-down and co-immunoprecipitation (Co-IP) assays showed that there were interactions among BnaA9.NF-YA7, BnaA9.NF-YB2, and BnaA6.NF-YC4 in vitro and in vivo (Fig. 5c, d ). EMSA also revealed band shifts when BnaA9.NF-YA7, BnaA9.NF-YB2, and BnaA6.NF-YC4 were all present (Fig. 5e and Supplementary Fig. 18d ). Interestingly, the dual-luciferase reporter assay showed that neither BnaA9.NF-YA7 G - nor BnaA9.NF-YA7 C -related trimers significantly induced the LUC activity of Bna . ABF3/4 reporters (Supplementary Fig. 18e ). Therefore, we speculated that BnaA9.NF-YA7 -related trimers participate in Bna.ABF3/4 -mediated regulatory pathways in an unknown way. To test this hypothesis, we examined the expression of downstream genes of BnaABF3s and BnaC1.ABF4 in WT, BnaA9.NF-YA7-OE, and BnaA9.NF-YA7-KO. RT‒qPCR analysis showed that the transcript levels of these downstream genes were significantly downregulated in BnaA9.NF-YA7-OE and slightly upregulated in BnaA9.NF-YA7-KO compared to WT under drought stress (Supplementary Fig. 19 ). These results suggest that BnaA9.NF-YA7 represses the BnaABF3/4 -regulated pathway through trimerization in response to drought stress. Next, we further analyzed the downstream target gene BnaC7.ABF3 , which is an upstream regulatory factor of BnaA9.NF-YA7 . In comparison with the WT, overexpression of BnaC7.ABF3 alone significantly increased survival because of increased leaf water holding capacity and decreased transpiration and water loss rates (Fig. 5f–h and Supplementary Fig. 20 ). In contrast, RNAi silencing of BnaC7.ABF3 , led to a similar phenotype as that of the BnaA9.NF-YA7-OE lines that showed increased sensitivity to drought stress, while co-overexpression of BnaA9.NF-YA7 and BnaC7.ABF3 led to an intermediate phenotype (Fig. 5f and Supplementary Fig. 20 ). These results suggest that there may be a negative feedback regulatory loop between BnaA9.NF-YA7 and BnaC7.ABF3 . BnaA9.NF-YA7 regulates drought responses via regulation of the H3K36me3 status Previous studies have established a correlation between NF-Y binding and posttranslational modifications, particularly histone modifications [16] , [21] , [22] , [23] , [24] . To examine the specific methyltransferase activities of BnaA9.NF-YA7 , the histone modification status was detected using specific antibodies through western blotting, and H3K36me3 levels were found to be specifically increased in the knockout lines and reduced in the overexpression transgenic lines compared with those of the WT (Fig. 6a, b ). RNA-Seq and RT-qPCR showed that BnaA9.NF-YA7 could repress Bna.ASHH4s expression, which encodes a histone-lysine N-methyltransferase involved in histone H3K36 methyltransferase activity (Fig. 6c ). Correspondingly, ChIP analysis of H3K36 trimethylation at the BnaC1.ABF3 and BnaC7.ABF3 loci in different genotypes revealed that overexpression of BnaA9.NF-YA7 significantly reduced the extent of H3K36 trimethylation at BnaC1.ABF3 and BnaC7.ABF3 (Fig. 6d , e). Comparable changes were not observed in chromatin at the BnaA2.ACT7 locus, which was used as a negative control (Supplementary Fig. 21a ). Next, we performed virus-induced Bna.ASHH4s silencing using a tobacco rattle virus (TRV)-based system to reduce Bna.ASHH4s mRNA levels and determined the expression level of BnaC1.ABF3 and BnaC7.ABF3 in TRV2-Bna.ASHH4 plants. The results indicated that BnaC1.ABF3 and BnaC7.ABF3 expression were positively correlated with Bna.ASHH4s expression. The expression of BnaC1.ABF3 and BnaC7.ABF3 in TRV2-Bna.ASHH4 plants did not significantly increase even under dehydration conditions (Supplementary Fig. 21b ). In turn, H3K36 trimethylation at BnaC1.ABF3 and BnaC7.ABF3 showed significant reduction in the TRV2-Bna.ASHH4 lines (Supplementary Fig. 21c ). The expression level of BnaA9.NF-YA7 was not affected by the downregulation of Bna.ASHH4s under normal conditions. Moreover, ChIP analysis of H3K36 trimethylation in Hap3 and Hap4 genotypes revealed that high expression level of BnaA9.NF-YA7 significantly reduced the extent of H3K36 trimethylation at BnaC1.ABF3 and BnaC7.ABF3 loci but not BnaA4.DOR and BnaA2.ACT7 loci (Supplementary Fig. 22 ). Taken together, these results indicate that BnaA9.NF-YA7 suppresses the expression of BnaABF3s by indirect regulation by H3K36me3 via Bna.ASHH4s . Fig. 6: BnaA9.NF-YA7 regulates drought responses via regulation of the histone H3 lysine 36 trimethylation (H3K36me3) status of the BnaABF3s locus. a Examination of H3K36 methyltransferase activity. Equal amounts of total proteins extracted from the nuclei of the wild-type (WT), BnaA9.NF-YA7 knockout lines (KO-2#, KO-7#, and KO-9#), and BnaA9.NF-YA7 overexpression lines (OE-7#, OE-8#, and OE-16#) were used for western blotting assays using different histone methylation antibodies, with H3 antibody as a loading control. b Relative protein levels in the WT, BnaA9.NF-YA7 knockout lines, and BnaA9.NF-YA7 overexpression lines. The amount of protein was determined by first normalizing the band intensity of specific antibodies using ImageJ software. c Genome browser view of RNA-Seq tags from the RNA-Seq data and RT-qPCR show that Bna.ASHH4s , which encodes a histone-lysine N-methyltransferase involved in histone H3K36 methyltransferase activity, repressed by BnaA9.NF-YA7 . The values are means ± SD ( n = 3 biological replicates). d , e BnaA9.NF-YA7 regulates H3K36me3 levels at the BnaC1.ABF3 locus ( d ) and B naC7.ABF3 locus ( e ) under drought stress. ChIP‒qPCR was performed using an H3K36me3 antibody. The x-axis denotes different genetic regions of BnaC1.ABF3 ( d ) and BnaC7.ABF3 ( e ). The values are means ± SD ( n = 3 biological replicates). Source data are provided as a Source Data file. Full size image BnaA9.NF-YA7 inhibits ABA-induced stomatal closure via upregulating BnaA4.DOR expression Among these common DEGs, BnaA4.DOR , which encodes the F-box protein DOR that functions as an inhibitory factor for ABA-induced stomatal closure under drought stress [25] , [26] , was significantly upregulated in the BnaA9.NF-YA7-OE lines but barely expressed in the other genotypes (Supplementary Fig. 19 ). ChIP-Seq and EMSA showed that BnaA9.NF-YA7 could bind the BnaA4.DOR promoter in vivo and in vitro (Fig. 7a, b ). However, ChIP analysis of H3K36 trimethylation at the BnaA4.DOR locus in different genotypes showed no significant change in the extent of H3K36 trimethylation at BnaA4.DOR (Supplementary Figs. 21a and 22 ). The expression level of BnaA4.DOR in Hap3 was significantly higher than that in Hap4 (Fig. 7c ). Transient expression assays confirmed that co-expression of BnaA9.NF-YA7 G with the NF-YB/C dimer induced higher LUC activity of the pBnaA4.DOR reporter than co-expression of BnaA9.NF-YA7 C with NF-YB/C dimer (Fig. 7d ). To further determine the role of BnaA4.DOR in BnaA9.NF-YA7-OE mediated drought sensitivity, we performed virus-induced BnaA4.DOR silencing using a TRV-based system to reduce BnaA4.DOR mRNA levels in BnaA9.NF-YA7-OE leaves (Fig. 7e ). Most TRV2-BnaA4.DOR plants survived after a subsequent 5-day recovery by watering. Although the survival rate was still lower than that of the WT, it was much higher than that of BnaA9.NF-YA7-OE plants (Fig. 7e , f). The water loss rate was significantly lower in BnaA4.DOR-silenced plants than in control plants (Fig. 7g ). Furthermore, the percentage of closed stomata was significantly higher in TRV2-BnaA4.DOR plants (46.80%) compared to control plants (30.75%) (Fig. 7h ) and exhibiting reduced stomatal conductance and a lower transpiration rate under nonstress conditions (Fig. 7i, j ). These results may explain why overexpression of BnaA9.NF-YA7 increases ABA sensitivity but does not significantly induce stomatal closure. Fig. 7: BnaA9.NF-YA7 induces BnaA4.DOR under drought stress, thereby increasing the rate of water loss. a Genome browser view of normalized ChIP-seq tags from the ChIP-seq data and normalized RNA-seq tags from the RNA-seq data for BnaA9.NF-YA7 , showing that BnaA4.DOR binds BnaA9.NF-YA7 . b EMSA showing that NF-Y containing BnaA9.NF-YA7 could bind the CCAAT sites in the BnaA4.DOR promoter. c Expression levels of BnaA4.DOR in Hap3 and Hap4 under normal conditions. The values are means ± SD ( n = 3 biological replicates). P values were calculated with the two-tailed Student’s t -test. d Co-expression of Bna.NF-YAs with the NF-YB/C dimer activate the expression of BnaA4.DOR . The values are means ± SD ( n = 3 biological replicates). The lowercase letters indicate significant differences ( P < 0.05, one-way ANOVA followed by a two-tailed LSD test). e Phenotyp e of BnaA4.DOR-silenced BnaA9.NF-YA7-OE plants. Four-week-old TRV2: BnaA4.DOR and TRV2:00 plants were exposed to drought stress by withholding watering for 10 days and rewatering for 2 days. Representative images and infrared thermal images were taken before and after drought stress and rewatering. White bars = 5 cm. f Survival rates of plants after rewatering. The values are means ± SDs ( n = 50 pla n ts examined over five independent experiments). P values were calculated with the two-tailed Student’s t -test. g The water holding capacity of TRV2: BnaA4.DOR and TRV2:00 leaves. The values are means ± SD ( n = 10 biologically independent plants in TRV2; n = 30 biologically independent plants in TRV2: BnaA4.DOR). P values were calculated with the two-tailed Student’s t -test. h Stomata type (%) in TRV2: BnaA4.DOR and TRV2:00 leaves under normal conditions. The values are means ± SD ( n = 10 biologically independent experiments). P values were calculated with the two-tailed Student’s t -test. i , j Stomatal conductance ( i ) and transpiration rate ( j ) in TRV2: BnaA4.DOR and TRV2:00 leaves under normal conditions. The values are means ± SD ( n = 10 biological replicates in TRV2; n = 20 biological replicates in TRV2: BnaA4.DOR). P values were calculated with the two-tailed Student’s t -test. Source data are provided as a Source Data file. Full size image Natural variation in functional genes play extremely important roles in crop trait divergence. In rice, two SNPs in the coding region of NRT1.1B contribute to higher nitrogen-use efficiency and improved grain yield [27] . A tandem repeat of the CCATTC sequence in the OsSPL13 5′ UTR causes reduced expression levels of OsSPL13 and results in small grains [28] . In maize, a 366-bp insertion in the promoter of ZmVPP1 contributes significantly to drought tolerance [29] . A two-base sequence polymorphism in UPA2 was associated with the different binding affinities of DRL1 , and the wild-type UPA2 allele showed narrow leaf angles and promoted yield under high-density planting in maize [30] . Natural variation in ZmFBL41 confers resistance to Rhizoctonia solani , that two amino acid substitutions prevent its interaction with ZmCAD , resulting in the inhibition of ZmCAD degradation and, consequently, the accumulation of lignin and the restriction of lesion expansion [31] . In cucumber, Che et al. identified a nonsynonymous polymorphism (G to A) in CsCRC as underlying the major effect of fruit size [32] . They found that CsCRC G , but not CsCRC A , targets the downstream auxin-responsive protein gene CsARP1 to regulate its expression [32] . These reports have confirmed that natural variations and their favorable alleles can be utilized as important genetic resources for trait improvement in crop breeding. Here, we found that a nonsynonymous polymorphism (G to C, M63I) and deletion of the CCAAT-box of the promoter in BnaA9.NF-YA7 affects the drought tolerance of B. napus . The accessions with the BnaA9.NF-YA7 C allele had a higher WHC than the accessions with the BnaA9.NF-YA7 G allele under drought treatment. The materials carrying the C allele were further divided into two types (Hap1 and Hap4), and Hap4 had stronger drought tolerance than Hap1 (Supplementary Fig. 5c ). However, deletion of the CCAAT-box, which reduced the BnaA9.NF-YA7 expression level, occurred only in Hap4, suggesting that the M63I substitution cooperates with CCAAT-box deletion and can be used to increase the drought tolerance of B. napus . Crops, including B. napus , exist in constantly changing environments and are often exposed to large amounts of abiotic and biotic stresses during their lifecycle. Among these stresses, drought stress is one of major environmental factors affecting the geographical distribution of plants in nature, limiting crop productivity in agriculture, and threatening food security [33] . The ABA signaling pathway is central to drought- and salt-stress responses in plants [34] . ABFs are known as master regulators of ABA signaling in response to drought and osmotic stresses, and the activation of genes containing an ABA-responsive element (ABRE) is largely dependent on ABF transcription factors [20] , [35] , [36] . In the presence of ABA, the activation of SnRK2s leads to the phosphorylation of ABF proteins, thus allowing ABFs to induce the expression of other ABA-responsive genes [20] , [37] . In this study, we found that fluridone (FLU) inhibited the upregulated expression of BnaA9.NF-YA7 induced by ABA treatment (Supplementary Fig. 5f ), and ABFs directly regulated BnaA9.NF-YA7 expression (Fig. 4 ), suggesting that BnaA9.NF-YA7 may also mediate the regulation of the drought response via an ABA-dependent pathway. Under stress conditions, the activation of ABA signaling helps plants respond to environmental stress and thus help them survive under adverse conditions. However, overexpression of drought-responsive genes often results in growth deficits and yield loss [38] . Therefore, balancing ABA signaling is very important for plants’ ability to cope with the changing environment [39] . Studies on switching off ABA signaling have mostly focused on the genes of the PYL-PP2C-SnRK2 pathway, which is the core pathway of ABA signal transduction, and few reports have focused on ABFs and their downstream genes. In this study, we found that the NF-Y complex involving BnaA9.NF-YA7 specifically binds to the promoter and CDS of BnaABF3s and reduces histone H3 Lys 36 (H3K36) trimethylation levels to inhibit their expression, thus attenuating ABA signaling (Figs. 5 and 6 ). These results suggest that the negative feedback regulatory network mediated by BnaA9.NF-YA7 serves as a supplementary mechanism for ABA signal balance. Stomatal closure preserves water in the plant, and ABA has a role in the regulation of stomatal movement to prevent water loss [40] . Because stomatal movements control CO 2 influx and transpiration, drought tolerance strategies to reduce water loss via stomatal closure occur at the expense of photosynthesis, growth, and yield [38] . 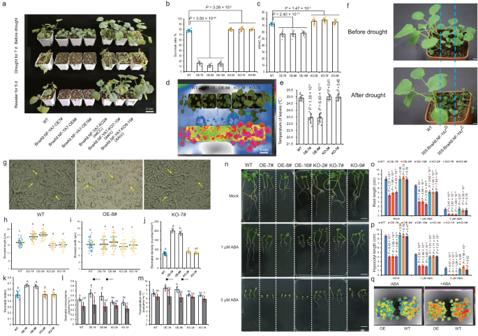Fig. 2:BnaA9.NF-YA7negatively regulatesB. napusdrought tolerance by increasing stomatal conductance and the transpiration rate. aPhenotype ofB. napusseedlings grown in plastic pots under well-watered, drought stress, or rewatering conditions. Bar = 5 cm.b,cThe survival rate (b) and water holding capacity (c) of overexpression and knockout lines were compared with those of WT. The values are means ± SD (n= 50 plants examined over ten independent experiments in (b) andn= 10 biologically independent experiments in (c).Pvalues were calculated with the two-tailed Student’st-test.d,eInfrared thermal images show the wild-type andBnaA9.NF-YA7transgenic lines (d) and the corresponding leaf surface temperature (e) before drought treatment. The values are means ± SD (n= 10 biologically independent experiments).Pvalues were calculated with the two-tailed Student’st-test. Bar = 5 cm.fThe drought tolerance was not significantly different between the 35S:BnaA9.NF-YA7Cand 35S:BnaA9.NF-YA7Gtransgenic lines. Bar = 1 cm.gPhenotype of stomata between wild-type andBnaA9.NF-YA7transgenic lines under well-watered conditions. Bar = 10 μm.h–kComparison of stomatal length (h), stomatal width (i), stomatal density (j), and stomatal index (k) between wild-type andBnaA9.NF-YA7transgenic lines. The values are means ± SD (n= 50 biological replicates in (h,i);n= 10 biological replicates in (j,k).l,mStomatal conductance (l) and transpiration rate (m) before and after ABA treatment. Values are mean ± SD (n= 5 biologically independent experiments). The lowercase letters indicate significant differences (P< 0.05, One-way ANOVA followed by two-tailed LSD test).nPhenotype of different genotypes grown on half-strength MS phytoagar medium containing 0, 1, or 5 μM ABA for 14 days under LD conditions. White bars = 2 cm.o,pQuantification of root length (o) and hypocotyl length (p) after 14 days of ABA treatment. The values are means ± SDs (n= 10 biological replicates).Pvalues were calculated with the two-tailed Student’st-test.qInfrared thermal images of WT and BnaA9.NF-YA7-OE plants before and after ABA treatment. White bars = 1 cm. Source data are provided as a Source Data file. Here, we found that overexpression of BnaA9.NF-YA7 increased ABA sensitivity, but the percentage of closed stomata was not significantly affected by ABA (Fig 21-q). We propose that this strategy may be part of an ABA signaling balance mechanism. BnaA9.NF-YA7 and its NF-Y complexes directly interact with the BnaA4.DOR promoter upregulates its expression level, thereby maintaining partial stomatal opening under drought stress and ensuring the CO 2 influx needed for plant photosynthesis, allowing plants to continue to grow under drought stress conditions. The M63I substitution occurred in a Pro-rich transcriptional activation domain, resulting in a transcriptional activation difference between BnaA9.NF-YA7 G and BnaA9.NF-YA7 C (Fig. 7d ), thus breaking the fine-tuning of the balance between opening and closing stomata under drought stress. Nevertheless, the impact of the M63I mutation on drought tolerance is limited and only when accompanied by the CCAAT mutation can it further enhance drought tolerance. This may also explain why Hap4 exhibits stronger drought tolerance than Hap1 (Fig. 1c, d ). Therefore, we posit that these two mutations are both independent yet intricately linked, with CCAAT primarily influencing the feedback regulation loop, while M63I predominantly modulates stoma sensitivity toward ABA. The excessive expression of BnaA9.NF-YA7 G/C excessively inhibited the transmission of ABA signals, and although the overexpression of BnaA9.NF-YA7 C promotes stomatal closure, it is insufficient to reverse the drought sensitivity caused by the inhibition of ABA signaling (Fig. 2f ). Taken together, the data indicate that BnaA9.NF-YA7 plays a dual role as both an inhibitor and activator, effectively regulating ABA signaling in rapeseed to maintain a balance between growth and drought stress responses. In summary, we propose the following hypothesis for how the drought tolerance difference between Hap4 and other haplotypes is regulated (Fig. 8 ): the expression of ABF genes and the accumulation of ABF proteins are induced by ABA signaling under drought stress, thus allowing ABFs to induce the expression of BnaA9.NF-YA7 and other ABA-responsive genes. The upregulated BnaA9.NF-YA7 can regulate the cascade strength of ABA signaling by reducing the H3K36me3 level to indirectly inhibit the expression of BnaABF3/4s , and thus BnaABF3/4s and BnaA9.NF-YA7 forms a regulatory loop to prevent excessive amplification of ABA signaling, thereby maintaining the dynamic balance between growth and the stress response in B. napus . Compared with the other haplotypes, Hap4, containing a two-base sequence variant (CCAAT-box deletion) at the promoter, is associated with a lower binding affinity for NF-Y. Low BnaA9.NF-YA7 expression in Hap4 and differences in transcriptional activation produced by the M63I substitution result in higher BnaABF3/4 s levels and a lower BnaA4.DOR level, consequently decreasing the transpiration rate and water loss rate and increasing the leaf water holding capacity. Although the contribution of BnaA9.NF-YA7 alone to improve B. napus drought tolerance was limited, our findings provide prospective drought tolerance allele. Furthermore, we add insights into the mechanisms that control ABA signaling homeostasis. Fig. 8: Working model demonstrating how the drought tolerance difference between Hap4 and other haplotypes is regulated at the molecular level. All haplotypes except Hap4 are collectively referred to as BnaA9.NF-YA7 Hap . Arrows indicate upregulation, and lines ending with bars represent downregulation. The thickness of the lines represents the strength of the regulation. The BnaABF3/4 proteins promote the upregulation of BnaA9.NF-YA7 expression by direct DNA-binding at its promoter region under drought stress. To prevent excessive amplification of the ABA signal, the upregulated BnaA9.NF-YA7 regulates the cascade strength of the ABA signal by reducing the H3K36me3 level to inhibit the expression of BnaABF3/4s . On the other hand, BnaA9.NF-YA7 negatively regulates drought tolerance by promoting BnaA4.DOR activity via direct DNA binding at its promoter region. Hap4 containing a two-base sequence variant (CCAAT-box deletion) at the promoter is associated with a lower binding affinity for NF-Y than the other haplotypes. Low BnaA9.NF-YA7 expression in Hap4 and differences in transcriptional activation produced by the M63I substitution result in high BnaABF3/4s levels and low BnaA4.DOR level, consequently decreasing the transpiration rate and water loss rate and leading to stronger drought resistance. Full size image Plant materials The diversity panel used in this study was from a previous report [18] . The B. napus transgenic lines used in this study were in the Zhongshuang 11 (ZS 11, Hap3) genetic background. The ProBnaA9.NF-YA7 :GUS transgenic line harboring a 1697 bp BnaA9.NF-YA7 promoter fragment was transformed into Arabidopsis (Col-0) by floral dipping. Association analysis A total of 205 overlapping lines from previous reports of Tan et al. and Lu et al. were used for association analysis of WHC [17] , [18] . The GWAS was conducted using the mixed linear model (MLM) [41] with a total of 581,532 SNPs (miss data <20%, MAF >0.05) in the GAPIT R package [42] . The Manhattan plot was displayed using the CMplot R package [43] . Phylogenetic analysis of BnaA9.NF-YA7 The full-length amino acid sequence of BnaA9.NF-YA7 was used for a BLAST search of the NCBI database ( http://www.ncbi.nlm.nih.gov/ ) to identify homologous genes in Brassicae species. The amino acid sequences were aligned using ClustalX 2.1 software. A phylogenetic tree was constructed using the neighbor-joining method with bootstrapping (1000 replicates) in MEGA version 5 [44] . Plasmid construction and B. napus transformation The BnaA9.NF-YA7 overexpression construct was generated with pENTR™ Directional TOPO® Cloning Kits (Invitrogen, USA) according to the manufacturer’s protocols, and the relevant fragment was cloned and inserted into the binary vector pEarleyGate 101. For BnaC7.ABF3 overexpression, the full-length CDS of BnaC7.ABF3 without the stop codon was amplified and cloned between the Bam HI and Sal I enzyme sites of the expression vector to generate the 35S:BnaC7.ABF3-DsRed fusion plasmid. The recombinant plasmids were introduced into the B. napus cultivar ZS 11 through Agrobacterium -mediated transformation. The transgenic plants were verified by PCR, and the expression levels in the transgenic plants were confirmed by RT-qPCR. For BnaA9.NF-YA7 knockout, two 18-bp targeting sequences were selected within the BnaA9.NF-YA7 and BnaC5.NF-YA7 gene. The sequences were synthesized and inserted into the p2×35S-dpCas9-atU6-Grna-35S-Hy vector to produce the CRISPR‒Cas9 plasmid. The CRISPR‒Cas9 plasmid was introduced into the B. napus cultivar ZS 11 through Agrobacterium-mediated transformation. The target was amplified by PCR using primer pairs flanking the designed target site, and the PCR product was sequenced. For the RNA interference (RNAi) construct, a unique 187-bp fragment from the cDNA of BnaA9.NF-YA7 was amplified and cloned between the Bam HI and Xba I enzyme sites of the pFGC5941M vector, and the antisense fragment was cloned into between the Nco I and Aat II enzyme sites of the pFGC5941M vector to form a hairpin structure. A unique 191-bp fragment from the cDNA of BnaC7.ABF3 was amplified and cloned into the pFGC5941M vector. The recombinant plasmids were introduced into the B. napus cultivar ZS 11 through Agrobacterium -mediated transformation. The transgenic plants were verified by PCR, and the expression levels in the transgenic plants were confirmed by RT-qPCR. For VIGS (virus-induced gene silencing), a unique 331-bp fragment from the cDNA of BnaA4.DOR and a unique 212-bp fragment from the cDNA of Bna.ASHH4 were amplified and reverse-cloned between the Bam HI and Eco RI enzyme sites of the pTRV2 vector, respectively. pTRV1 and pTRV2 were transformed into Agrobacterium tumefaciens (strain GV3101) and subsequently used for the infection of B. napus seedlings. For site-directed mutagenesis, the site-directed mutation of the 189th base of Hap3 (G to C) was achieved by overlap extension PCR, followed by cloning the relevant fragment into the binary vector pCAMBIA1302 to create pBnaA9.NF-YA7 H3 :Hap3, pBnaA9.NF-YA7 H4 :Hap4, and pBnaA9.NF-YA7 H3 :Hap3 C constructs, respectively. Transgenic Arabidopsis plants were generated through floral-dip by Agrobacterium -mediated transformation. Stress treatment and physiological experiments To assess the drought stress tolerance of WT and transgenic plants, 7-day-old seedlings were transferred to pots, grown for 3 weeks under normal conditions, and subjected to drought conditions by withholding water from the seedlings for 1 week, 10 days, or 14 days [45] . The drought-related phenotypes were photographed with a camera (DS126611, Canon). The leaf water loss rate and relative water content (RWC) were determined as previously described by refs. [8] , [46] . Briefly, at least five leaves from different plants of each genotype were detached from 3-week-old plants and placed in a petri dish on a laboratory bench (22 ± 1 °C and 30–40% RH), and the weight of the detached leaves was then measured every 1 h for a period of 48 or 12 h. The experiment was repeated three times. Water loss was presented as the percentage of initial water loss. For the RWC, the leaves were detached from 3-week-old plants and weighed to obtain leaves weight (W), after which the leaves are immediately hydrated to full turgidity for 12 h under normal room light and temperature. After hydration, the leaves are weighed to obtain fully turgid weight (TW). Leaves are then oven-dried at 85 °C for 24 h and weighed to determine dry weight (DW). The relative water content was calculated using the following formula: 
    RWC(%)=[(W-DW)/(TW-DW)]× 100
 (1) To measure water holding capacity (WHC), fully expanded fourth leaves were detached from the seedlings, and the petioles were wrapped with fresh-keeping film to prevent water loss from the petioles. The fresh weight of detachment leaves was measured immediately detached from the plants (W f ), 24 h dark treatment (23 ± 1 °C and 30–40% RH, W t ), and drying (W d ). The water holding capacity of separated leaves was calculated using the following formula shown as percentage: 
    WHC(%)=(W_t-W_d)/(W_f-W_d)× 100
 (2) The experiment was repeated three times. For each repeat, at least five leaves from different plants of each genotype were used. The soluble protein content was determined by the Coomassie Brilliant Blue G250 method, and the free proline content was measured by the sulfosalicylic acid colorimetric method [47] , [48] . For the stomatal aperture assay, epidermal strips were peeled from 4-week-old plants, and the mesophyll cells were removed with a small brush [45] , For the ABA-mediated stomatal closure assay, the leaves were incubated in MES buffer (10 mM MES-KOH, pH 6.15, 10 mM KCl, and 50 mM CaCl 2 ) in light for 3 h at 22 °C to open the stomata. After the addition of 20 mM ABA or DMSO (control) to the buffer and incubation of the leaves for an additional 2 h, images were taken by an optical microscope equipped with a digital camera (Nikon ECLIPSE E600, Japan). The stomatal aperture was analyzed using ImageJ software, and three independent repeats were performed. Histochemical GUS staining and GUS activity The promoter sequence of BnaA9.NF-YA7 was amplified from ZS 11 (Hap3) and R219 (Hap4) and inserted into the binary vector pCAMBIA1305.1 to create pBnaA9.NF-YA7 Hap3 :GUS and pBnaA9.NF-YA7 Hap4 :GUS reporter gene constructs, respectively. For promoter truncation, differently truncated promoters of BnaA9.NF-YA7 were amplified and cloned between the Xba I and Nco I enzyme sites of the pCAMBIA1305.1 vector to generate promoter :GUS fusion plasmids. The recombinant plasmids were transformed into Arabidopsis (Col-0) by floral dipping. For the positive lines, plants from the T3 generation were used for GUS staining, which was performed according to the method described in the manufacturer’s protocols for the GUS Staining Kit (Coolaber, China). The stained tissues were photographed by an optical microscope equipped with a digital camera (Nikon SMZ1500, Japan). GUS activity was measured by the fluorometry method [49] . RNA extraction, qRT–PCR, and RNA-sequencing Total RNA was extracted from 4-week-old seedlings before and after drought treatment with an EZ-10 DNAaway RNA Mini-Prep Kit (Sangon Biotech, China) according to the manufacturer’s protocols. For RT‒qPCR, cDNA was synthesized from the total RNA using a PrimeScript TM RT reagent kit with gDNA Eraser (TaKaRa, Japan) as described in the supplier’s instructions. RT‒qPCR analyses were performed with TB Green® Premix Ex Taq™ II (Takara) on a CFX96 Real-Time PCR Detection System. PCR amplification was performed with a 3 min denaturing step at 95 °C, followed by 40 cycles of 95 °C for 15 s and 60 °C for 30 s. Three independent biological replicates were collected for each sample. Bna.Actin7 was used as the internal control. The comparative CT (2 -ΔCT ) method [50] was used to quantify the relative gene expression levels. For RNA-Seq, total RNA was extracted from B. napus leaves of Hap3, Hap4, WT, BnaA9.NF-YA7-OE, and BnaA9.NF-YA7-KO lines before and after drought treatment. High-quality RNA was sent to Biomarker Technologies Co., Ltd. (Beijing, China) for sequencing and analysis. TopHat2 software was used for reference genome (Darmor-bzh v4.1) mapping. Visualize the alignment results of Reads on the genome using IGV software. Transcript abundance was calculated as fragments per kilobase of transcript per million mapped reads (FPKM) values. Differentially expressed genes (DEGs) of two conditions/groups was performed using the DESeq2. The resulting P values were adjusted using Benjamini and Hochberg’s approach for controlling the false discovery rate. Genes with an adjusted P -value < 0.05 found by DESeq2 were assigned as differentially expressed. The FDR <0.05 and fold change ≥1.5 was set as the threshold for significantly differential expression. Thermal imaging Thermal imaging of plants was performed as described previously with some modifications [45] . Briefly, the plants were grown at 20 to 22 °C under a 16-h-light/8-h-dark cycle in a greenhouse for 4 weeks. Water was then withheld for 1 week before measurements. Thermal images were obtained using a WIC640 infrared camera (Workswell, Czech Republic). Leaf temperature was measured using Workswell CorePlayer professional software. For each genotype, plants in three different pots were analyzed, with similar results. Yeast one-hybrid, two-hybrid, and three-hybrid assays An approximately 0.5 kb core promoter DNA fragment of BnaA9.NF-YA7 was inserted upstream of the AbA r reporter gene in the pAbAi vector as the pBait-AbAi plasmid. A B. napus cDNA library was prepared in the pGADT7-Rec vector in the Matchmaker® Gold Yeast One-Hybrid Library Screening System (PT4087-1, Clontech, USA) using RNA isolated from 4-week-old seedlings after drought stress treatment according to the manufacturer’s instructions. Yeast one-hybrid screening and one-hybrid interaction assays were performed by the user manual supplied with the Matchmaker Gold Yeast One-Hybrid Library Screening System (PT4087-1, Clontech, USA). For the yeast two-hybrid assay (Y2H), the full-length BnaA9.NF-YA7 coding sequence was cloned and inserted into the Eco RI and Bam HI sites of the prey vector pGADT7 or into the Eco RI and Bam HI sites of the bait vector pGBKT7. The full-length CDSs of BnaNF-YB genes and BnaNF-YC genes were cloned and inserted into the pGADT7 and pGBKT7 vectors, respectively. The coding region of BnaC7.ABF3 was amplified and inserted into pGADT7 as AD-BnaC7.ABF3 and BnaA3.ABF4 was amplified and inserted into pGBKT7 as BD-BnaA3.ABF4. For interaction assays, the specific bait and prey constructs were co-transformed into yeast Y2HGold cells using the Yeastmaker TM Yeast Transformation System 2 (PT1172-1, Clontech, USA) according to the manufacturer’s instructions and grown on SD/-Trp/-Leu and SD/Trp/-Leu/-His/-Ade media for interaction tests. For the yeast three-hybrid assay (Y3H), the pBridge vector was used to express both BnaNF-YBs and BnaNF-YCs. The pGADT7 vector was used to express BnaNF-YAs, BnaC7.ABF3 , and BnaA3.ABF4 . Moreover, the BnaA9.NF-YB2 coding sequence was cloned and inserted into the Eco RI and Bam HI sites of multiple cloning site I (MCSI) and the BnaA6.NF-YC4 coding sequence was cloned and inserted into the Not I and Bgl II sites of MCSII of the pBridge vector as a bait plasmid. A B. napus cDNA library was prepared in the pGADT7-Rec vector in the Matchmaker® Gold Yeast Two-Hybrid Library Screening System (PT4084-1, Clontech, USA) using RNA isolated from 4-week-old seedlings after drought stress treatment according to the manufacturer’s instructions. Yeast three-hybrid screening and three-hybrid interaction assays were performed by the user manual supplied with the Matchmaker® Gold Yeast Two-Hybrid Library Screening System (PT4084-1, Clontech, USA). BiFC assay The coding regions of BnaNF-Ys were amplified and inserted into the pXY104 vector containing the C-terminus of yellow fluorescent protein (cYFP) and the pXY106 vector containing the N-terminus of yellow fluorescent protein (nYFP). The coding region of BnaC7.ABF3 was amplified and inserted into the pXY104 vector and the coding region of BnaA3.ABF4 was amplified and inserted into the pXY106 vector. 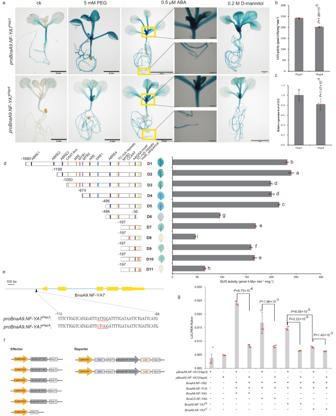Fig. 3: CCAAT-box variation affects the expression level ofBnaA9.NF-YA7. aGUS staining ofProBnaA9.NF-YA7Hap3:GUS andProBnaA9.NF-YA7Hap4:GUS seedlings under normal conditions and 5 mM PEG, 0.5 µM ABA, and 0.2 Md-mannitol treatment. Scale bars, 2 mm, 5 mm or 500 µm.b,cGUS enzyme activity (b) and GUS expression level (c) betweenProBnaA9.NF-YA7Hap3:GUS andProBnaA9.NF-YA7Hap4:GUS seedlings under normal conditions. The values are means ± SD (n= 3 biological replicates).Pvalues were calculated with the two-tailed Student’st-test.dGUS enzyme activity of transgenic plants after fusion of the GUS reporter gene withBnaA9.NF-YA7promoter fragments of different lengths. The values are means ± SDs (n= 3 biologically independent experiments). D1–D11 indicatesBnaA9.NF-YA7promoter fragments of different lengths. The lowercase letters indicate significant differences (P< 0.05, one-way ANOVA followed by a two-tailed LSD test).eSNP variation of the CCAAT-box within the promoter region ofBnaA9.NF-YA7between Hap4 and the other Haps. The sequences on the red lines are the target site. The red characters indicate substitutions.fSchematic diagram showing the constructs used in the transient transactivation analysis.gNF-Y trimers can activate the expression ofBnaA9.NF-YA7, and the CCAAT-box variation affects the expression level ofBnaA9.NF-YA7between Hap3 and Hap4. The values are means ± SD (n= 3 biologically independent experiments).Pvalues were calculated with the two-tailed Student’st-test. Source data are provided as a Source Data file. The plasmids were then transformed into Agrobacterium GV3101 cells with the silencing suppressor P19 strain. 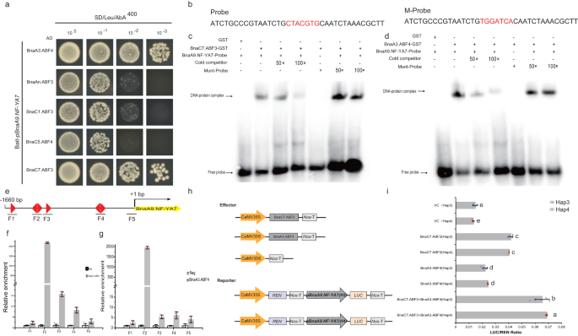Fig. 4:BnaABF3/4sdirectly upregulates the transcription ofBnaA9.NF-YA7. aY1H indicated that BnaABF3/4 s could bind theBnaA9.NF-YA7promoter.b–dEMSA showed that BnaC7.ABF3 (c) and BnaA3.ABF4 (d) could bind the ABRE sites in theBnaA9.NF-YA7promoter. The biotin-labeled probes are indicated in (b).eThe fragments used in ChIP‒qPCR.f,gChIP‒qPCR identified BnaC7.ABF3 (f) and BnaA3.ABF4 (g) as significantly enriched in the fragment containing the ABRE sites in theBnaA9.NF-YA7promoter. Fold enrichments in (f) and (g) were calculated relative to input. The values are means ± SD (n= 3 biological replicates).hSchematic diagram showing the constructs used in the transient transactivation analysis.iBnaC7.ABF3 and BnaA3.ABF4 activatesBnaA9.NF-YA7independently or in the form of dimers. The values are means ± SDs (n= 6 biologically independent experiments). The lowercase letters indicate significant differences (P< 0.05, One-way ANOVA followed by two-tailed LSD test). Source data are provided as a Source Data file. Then, these strains were resuspended in an induction medium (10 mM MES-KOH, pH 5.7, 10 mM MgCl 2 , 200 mM acetosyringone) to an OD 600 of 1.0. After incubation at room temperature for 3 h in darkness, the different strain combinations were mixed and infiltrated into Nicotiana benthamiana leaves. The plants were grown at 22 °C under a 12-h-light/12-h-dark cycle in a greenhouse for 48 to 72 h, and YFP signals were observed under a confocal laser-scanning microscope (Zeiss LSM 800). BiFC-FRET analysis For BiFC-based FRET analysis, the coding regions of BnaA9.NF-YB2 and BnaA6.NF-YC4 were cloned and inserted into the pXY106 vector and pXY104 vector to produce nYFP-BnaA9.NF-YB2 and cYFP-BnaA6.NF-YC4, respectively. The full-length sequences of BnaA9.NF-YA7 G and BnaA9.NF-YA7 C were amplified, and the N-terminus was fused to the CFP coding sequence, generating BnaA9.NF-YA7 G -CFP and BnaA9.NF-YA7 C -CFP, respectively. The plasmids were then transformed into Agrobacteria GV3101 cells with the silencing suppressor P19 strain. Then, Agrobacteria cultures containing equal amounts of nYFP-BnaA9.NF-YB2 and cYFP-BnaA6.NF-YC4 strains were mixed and infiltrated into Nicotiana benthamiana leaves to allow the formation of BiFC complexes (acceptors), along with equal amounts of BnaA9.NF-YA7 G -CFP or BnaA9.NF-YA7 C -CFP (donors) strain cultures. After infiltration, the plants were grown at 22 °C under a 12-h light/12-h dark cycle in a greenhouse for 48 to 72 h before analyses of interaction using FRET. An excitation wavelength of 458 nm and an emission wavelength of 470–500 nm was used for CFP, and an excitation wavelength of 514 nm and an emission wavelength of 515–545 nm were used for YFP. The FRET energy transfer efficiency was calculated using the following formula shown as percentage [51] , [52] : 
    E=(donor after-donor  before)× 100/donor  after
 (3) Pull-down assay The coding regions of BnaA9.NF-YB2-Myc , BnaA6.NF-YC4-His , BnaC7.ABF3 , BnaA3.ABF4 , BnaA9.NF-YA7 G , and BnaA9.NF-YA7 C were cloned and inserted into the pGEX-4T-1 vector to produce GST-BnaA9.NF-YB2-Myc, GST-BnaA6.NF-YC4-His, GST-BnaC7.ABF3, GST-BnaA3.ABF4, GST-BnaA9.NF-YA7 G , and GST-BnaA9.NF-YA7 C , respectively. The expression of GST recombinant proteins in E. coli Rosetta cells (DE3; TransGen Biotech, Beijing, China) was induced by treatment with 0.5 mM IPTG for 12 h. The proteins were purified using glutathione agarose beads (Beyotime Biotechnology, Beijing, China). The BnaA9.NF-YB2-Myc and BnaA6.NF-YC4-His proteins were obtained after the GST label was digested by thrombin following the manufacturer’s instructions. For the pull-down assay, equal amounts of BnaA9.NF-YB2-Myc and BnaA6.NF-YC4-His were incubated in binding buffer (50 mM Tris-HCl, pH 8.0, 100 mM NaCl, and 1 mM EDTA) with immobilized GST or GST-labeled proteins at 4°C for 4 h. The Glutathione agarose beads were then mixed with the protein mixture in 1 mL of PBS (140 mM NaCl, 2.7 mM KCl, 10 mM Na 2 HPO 4 , and 1.8 mM KH 2 PO 4 ) and mixed by rotation at 4 °C for 1 h. After washing three times with PBS, proteins that were retained on the beads were separated by SDS–polyacrylamide gel electrophoresis (PAGE). Western blot analysis was performed using anti-GST (1:2000), anti-Myc (1: 2000), and anti-His (1:2000) antibodies (Beyotime Biotechnology, Beijing, China). Co-IP assay The recombinant vectors (containing Myc-BnaA9.NF-YB2, His-BnaA6.NF-YC4, Flag-BnaC7.ABF3, Flag-BnaA3.ABF4, Flag-BnaA9.NF-YA7 G , and Flag-BnaA9.NF-YA7 C , respectively) were transformed into Agrobacterium tumefaciens strain GV3101 carrying p19 (35 S:p19). Then, these strains were resuspended in an induction medium to an OD 600 of 0.8. After incubation at room temperature for 3 h in darkness, the different strain combinations were mixed and infiltrated into N. benthamiana leaves. Total proteins were extracted from the samples with extraction buffer (50 mM Tris-MES (pH 8.0), 0.5 M sucrose, 1 mM MgCl 2 , 10 mM EDTA, 5 mM DTT, 1 mM PMSF, and 100× protease inhibitor cocktail) at 3 d.p.i and incubated with anti-Flag antibody immobilized onto Protein G/A-Agarose suspension (Beyotime Biotechnology, Beijing, China) in extraction buffer at 4 °C for 4 h. After incubation, the beads were washed with wash buffer (100 mM Tris-HCl (pH 8.0), 100 mM NaCl, and 1% [v/v] Triton X-100) and eluted with 5× SDS loading buffer. The proteins bound to the beads were resolved by SDS–PAGE and detected by anti-FLAG, anti-Myc, and anti-His antibodies (Beyotime Biotechnology, Beijing, China). Transient expression assay For the dual-luciferase transcriptional activity assays, the firefly luciferase (LUC) gene driven by the minimal TATA box of the CaMV 35S promoter following five copies of the GAL4 binding element was used as a reporter [53] . 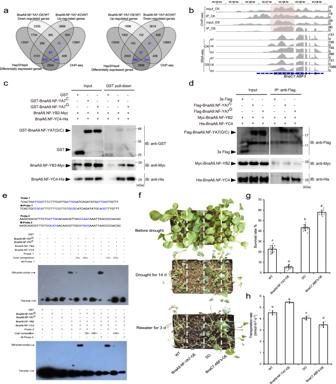Fig. 5:BnaA9.NF-YA7directly targetsBnaABF3s. aVenn diagrams of the DEGs from transcriptomes and target genes of ChIP-Seq.bGenome browser view of normalized ChIP-Seq tags from the ChIP-Seq data and normalized RNA-Seq tags from the RNA-Seq data forBnaA9.NF-YA7, showing examples ofBnaC7.ABF3bound byBnaA9.NF-YA7TFs.c,dGST pull-down (c) and co-immunicprecipitation assays (d) testing the interactions among BnaA9.NF-YA7 and BnaA9.NF-YB2/BnaA6.NF-YC4 in vitro and in vivo.eEMSA showing that NF-Y containing BnaA9.NF-YA7 could bind the CCAAT sites in theBnaABF3spromoter. Labeled probes containing the CCAAT element (Supplementary Fig.18d, near TSS or within the coding region) were synthesized and labeled with biotin. The cold (unlabeled) probe and mutated CCAAT element (labeled) were used as a competitor and mutant probes, respectively.fPhenotype ofB. napusseedlings grown in plastic bins (length × width × depth = 32 × 20 × 10 cm) under well-watered, drought stress, or rewatering conditions. WT indicates wild-type ZS 11 plants, DO indicatesBnaA9.NF-YA7andBnaC7.ABF3double overexpression lines Bar = 2 cm.gThe survival rate of BnaA9.NF-YA7-OE, BnaC7.ABF3-OE, and double overexpression lines were compared with that of the WT. The values are means ± SD (n= 50 plants examined over ten independent experiments).hTranspiration rate of BnaA9.NF-YA7-OE, BnaC7.ABF3-OE, and double overexpression lines were compared with WT under normal conditions. The values are means ± SD (n= 3 biological replicates). The lowercase letters indicate significant differences (P< 0.05, one-way ANOVA followed by a two-tailed LSD test). Source data are provided as a Source Data file. BnaA9.NF-YA7 CDS fragments of different lengths fused with the yeast GAL4 DNA-binding domain driven by the CaMV 35S promoter followed by the translational enhancer from tobacco mosaic virus were used as effectors [54] . For the dual-luciferase transient expression assays, the different promoter segments were recombined into the Hin dIII and Bam HI sites of the pGreenII 0800-LUC vector, generating the promoter :LUC plasmids as reporters. The Renilla luciferase (REN) gene driven by the 35S promoter in the pGreenII 0800-LUC vector was used as the internal control [30] . The full-length CDSs of different genes were amplified and recombined into the Bam HI and Eco RI sites of the pGreenII 62-SK vector driven by the 35S promoter, forming different effectors. The empty pGreenII 62-SK vector was used as a control. Transient dual-luciferase assays were performed in Arabidopsis protoplasts collected from the leaves of 4-week-old seedlings. The luciferase signal was detected using the Dual-Luciferase Reporter Assay System (Promega, USA) with a GloMax 20/20 Luminometer (Promega, USA). Relative LUC activity was calculated by normalizing LUC activity to REN activity [30] . Chromatin immunoprecipitation assay Chromatin immunoprecipitation (ChIP) assays were performed using an EpiQuik TM Plant ChIP kit (Epigentek) according to the user guide. Leaf tissues (1 g) before and after drought treatment were collected from 35S: BnaA9.NF-YA7 -GFP transgenic seedlings grown in pots for 4 weeks. An anti-GFP antibody (ab290; Abcam) was used to immunoprecipitate the sonicated DNA‒protein complexes containing BnaA9.NF-YA7 -GFP. The qualified chromatin fragments were sent to Novogene ( www.novogene.com/ ) for ChIP-Seq analysis. High-quality clean reads were mapped to the public B. napus genome Darmor-bzh v4.1 with default parameters using the Burrows–Wheeler Aligner (BWA) [55] . To determine whether BnaABF3/4 regulates and controls BnaA9.NF-YA7 , chromatin immunoprecipitation was performed using BnaC7.ABF3-Flag , BnaA3.ABF4-Flag , and empty vector transgenic plant leaves. Sonicated chromatin fragments were immunoprecipitated using an anti-Flag antibody (CST, 14793S). 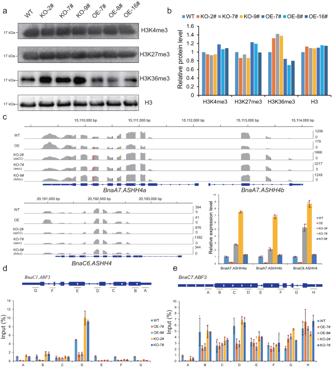Fig. 6:BnaA9.NF-YA7regulates drought responses via regulation of the histone H3 lysine 36 trimethylation (H3K36me3) status of theBnaABF3slocus. aExamination of H3K36 methyltransferase activity. Equal amounts of total proteins extracted from the nuclei of the wild-type (WT),BnaA9.NF-YA7knockout lines (KO-2#, KO-7#, and KO-9#), andBnaA9.NF-YA7overexpression lines (OE-7#, OE-8#, and OE-16#) were used for western blotting assays using different histone methylation antibodies, with H3 antibody as a loading control.bRelative protein levels in the WT,BnaA9.NF-YA7knockout lines, andBnaA9.NF-YA7overexpression lines. The amount of protein was determined by first normalizing the band intensity of specific antibodies using ImageJ software.cGenome browser view of RNA-Seq tags from the RNA-Seq data and RT-qPCR show thatBna.ASHH4s, which encodes a histone-lysine N-methyltransferase involved in histone H3K36 methyltransferase activity, repressed byBnaA9.NF-YA7. The values are means ± SD (n= 3 biological replicates).d,eBnaA9.NF-YA7regulates H3K36me3 levels at theBnaC1.ABF3locus (d) and BnaC7.ABF3locus (e) under drought stress. ChIP‒qPCR was performed using an H3K36me3 antibody. The x-axis denotes different genetic regions ofBnaC1.ABF3(d) andBnaC7.ABF3(e). The values are means ± SD (n= 3 biological replicates). Source data are provided as a Source Data file. For histone modification analysis, ChIP experiments were performed using WT, BnaA9.NF-YA7-OE, and BnaA9.NF-YA7-KO leaves. ChIP was performed using Protein A/G magnetic beads (ab193262; Abcam) and anti-H3K36me3 antibody (Abcam, ab9050), anti-H3K4me3 antibody (Abcam, ab8580), anti-H3K27me3 antibody (Abcam, ab6002), and anti-Histone H3 antibody (Abcam, ab1791). The precipitated DNA fragments were recovered and analyzed by RT‒qPCR using specific primers. 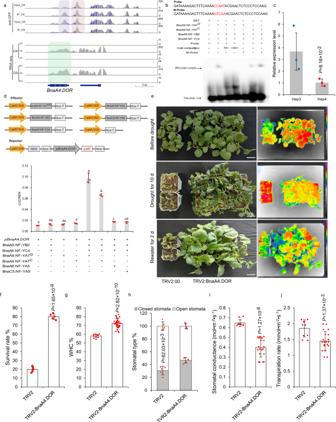Fig. 7:BnaA9.NF-YA7inducesBnaA4.DORunder drought stress, thereby increasing the rate of water loss. aGenome browser view of normalized ChIP-seq tags from the ChIP-seq data and normalized RNA-seq tags from the RNA-seq data forBnaA9.NF-YA7, showing thatBnaA4.DORbindsBnaA9.NF-YA7.bEMSA showing that NF-Y containing BnaA9.NF-YA7 could bind the CCAAT sites in theBnaA4.DORpromoter.cExpression levels ofBnaA4.DORin Hap3 and Hap4 under normal conditions. The values are means ± SD (n= 3 biological replicates).Pvalues were calculated with the two-tailed Student’st-test.dCo-expression of Bna.NF-YAs with the NF-YB/C dimer activate the expression ofBnaA4.DOR. The values are means ± SD (n= 3 biological replicates). The lowercase letters indicate significant differences (P< 0.05, one-way ANOVA followed by a two-tailed LSD test).ePhenotypeof BnaA4.DOR-silenced BnaA9.NF-YA7-OE plants. Four-week-old TRV2: BnaA4.DOR and TRV2:00 plants were exposed to drought stress by withholding watering for 10 days and rewatering for 2 days. Representative images and infrared thermal images were taken before and after drought stress and rewatering. White bars = 5 cm.fSurvival rates of plants after rewatering. The values are means ± SDs (n= 50 plants examined over five independent experiments).Pvalues were calculated with the two-tailed Student’st-test.gThe water holding capacity of TRV2: BnaA4.DOR and TRV2:00 leaves. The values are means ± SD (n= 10 biologically independent plants in TRV2;n= 30 biologically independent plants in TRV2: BnaA4.DOR).Pvalues were calculated with the two-tailed Student’st-test.hStomata type (%) in TRV2: BnaA4.DOR and TRV2:00 leaves under normal conditions. The values are means ± SD (n= 10 biologically independent experiments).Pvalues were calculated with the two-tailed Student’st-test.i,jStomatal conductance (i) and transpiration rate (j) in TRV2: BnaA4.DOR and TRV2:00 leaves under normal conditions. The values are means ± SD (n= 10 biological replicates in TRV2;n= 20 biological replicates in TRV2: BnaA4.DOR).Pvalues were calculated with the two-tailed Student’st-test. Source data are provided as a Source Data file. 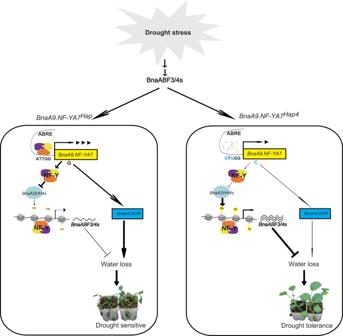Fig. 8: Working model demonstrating how the drought tolerance difference between Hap4 and other haplotypes is regulated at the molecular level. All haplotypes except Hap4 are collectively referred to asBnaA9.NF-YA7Hap. Arrows indicate upregulation, and lines ending with bars represent downregulation. The thickness of the lines represents the strength of the regulation. The BnaABF3/4 proteins promote the upregulation ofBnaA9.NF-YA7expression by direct DNA-binding at its promoter region under drought stress. To prevent excessive amplification of the ABA signal, the upregulatedBnaA9.NF-YA7regulates the cascade strength of the ABA signal by reducing the H3K36me3 level to inhibit the expression ofBnaABF3/4s. On the other hand,BnaA9.NF-YA7negatively regulates drought tolerance by promotingBnaA4.DORactivity via direct DNA binding at its promoter region. Hap4 containing a two-base sequence variant (CCAAT-box deletion) at the promoter is associated with a lower binding affinity for NF-Y than the other haplotypes. LowBnaA9.NF-YA7expression in Hap4 and differences in transcriptional activation produced by the M63I substitution result in highBnaABF3/4slevels and lowBnaA4.DORlevel, consequently decreasing the transpiration rate and water loss rate and leading to stronger drought resistance. ChIP‒qPCR assays were performed using three biological replicates and three technical replicates for each biological replicate. The fold enrichment was calculated against the GFP or Flag control samples. Reporting summary Further information on research design is available in the Nature Portfolio Reporting Summary linked to this article.